Immunochip SNP array identifies novel genetic variants conferring susceptibility to candidaemia Candidaemia is the fourth most common cause of bloodstream infection, with a high mortality rate of up to 40%. Identification of host genetic factors that confer susceptibility to candidaemia may aid in designing adjunctive immunotherapeutic strategies. Here we hypothesize that variation in immune genes may predispose to candidaemia. We analyse 118,989 single-nucleotide polymorphisms (SNPs) across 186 loci known to be associated with immune-mediated diseases in the largest candidaemia cohort to date of 217 patients of European ancestry and a group of 11,920 controls. We validate the significant associations by comparison with a disease-matched control group. We observe significant association between candidaemia and SNPs in the CD58 ( P =1.97 × 10 −11 ; odds ratio (OR)=4.68), LCE4A-C1orf68 ( P =1.98 × 10 −10 ; OR=4.25) and TAGAP ( P =1.84 × 10 −8 ; OR=2.96) loci. Individuals carrying two or more risk alleles have an increased risk for candidaemia of 19.4-fold compared with individuals carrying no risk allele. We identify three novel genetic risk factors for candidaemia, which we subsequently validate for their role in antifungal host defence. Candidaemia is the fourth most common bloodstream infection [1] , with known risk factors such as neutropenia, mucosal barrier injury, transplantation, immunosuppressive drugs, intravascular catheters and extended intensive care unit stay [2] , [3] , [4] . Despite the availability of potent antifungal drugs, the mortality of patients with candidaemia remains high (up to 37–44%) [5] , [6] . It has therefore been proposed that only intensified patient care, using risk assessment and adjuvant immunotherapy, may improve the outcome [7] . The host immune status is crucial for the outcome of Candida infections, and identifying genetic variation in immune genes that confer susceptibility to Candida infection may aid in designing effective preventive strategies. Several small-scale candidate gene association studies suggest a role in candidaemia risk for single-nucleotide polymorphisms (SNPs) in toll-like receptors ( TLR - 1 , TLR-2 , TLR-3 and TLR-4 ), interleukins (ILs) ( IL-12B and IL-10 ) and lymphoid protein tyrosine phosphatase PTPN22 (ref. 3 ). Interestingly, ~10 monogenic disorders have been reported to be associated with chronic mucocutaneous candidiasis, and almost all are caused by defects in genes of the immune system [3] . Intriguingly, common SNPs in 8 out of these 10 monogenic disorder genes ( AIRE , CARD9 , STAT1 , STAT3 , TYK2 , CD25 , IL17RA and IL17F ) are also associated with susceptibility to different immune-mediated diseases (NHGRI GWAS catalog [8] ), implying that genes necessary for immune regulation are strong candidates in determining susceptibility to fungal infections. Here we report the first genome-wide screen of ~200,000 SNPs in 186 loci in the largest candidaemia cohort to date. By using the Immunochip SNP array [9] , we identify three novel genetic risk factors for candidaemia that were validated using transcriptomics, pathway analysis and immunological studies. Association analysis identifies three candidaemia risk loci After filtering the Immunochip data using standard quality parameters, we obtained 118,989 SNPs from the 217 candidaemia cases and 11,920 healthy controls, which we analysed using logistic regression analysis. The results of this analysis revealed significant association ( P <5 × 10 −8 ) to three independent loci with candidaemia ( Fig. 1a ). 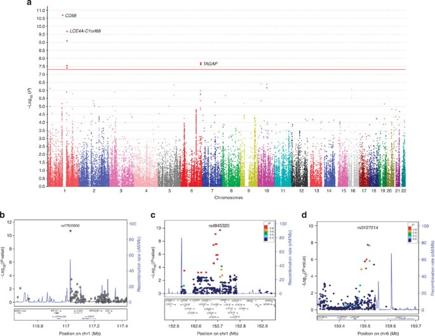Figure 1: Genetic association with candidaemia. (a) Manhattan plot showing the genome-widePvalues of association with candidaemia. Theyaxis represents the −log10Pvalues of 118,989 SNPs and their chromosomal positions are shown on thexaxis. The horizontal red line shows the genome-wide significant threshold ofP<5 × 10−8. TheP-values were obtained by logistic regression test after adjusting for the first four components from the multidimensional scaling analysis. Regional association plots at (b) 1p13.1, (c) 1q21.3 and (d) 6q25.3. ThePvalues of genotyped SNPs are plotted as –log10values against their physical chromosomal positions (hg19). Estimated recombination rates from the 1000 Genomes European population show the local LD structure. Inset, the colours of the SNPs indicate LD with the top-associated SNPs according to a scale fromr2=0 tor2=1 based on pairwiser2values from the 1000 Genomes European population. Lower panel, gene annotations from the University of California Santa Cruz genome browser (hg19). The top SNPs from these three loci were rare in healthy controls, with risk allele frequencies <2%, whereas the risk allele frequencies were >5% in candidaemia cases ( Table 1 ). The top-associated SNP, rs17035850 ( P =1.97 × 10 −11 ; odds ratio=4.68), is located in a block of linkage disequilibrium (LD) of ~30 kb at 1p13.1, which contains the CD58 gene ( Fig. 1b ), two long non-coding RNAs (lncRNA), RP5-1086K13.1 and RP4-655J12.4, and the pseudogene NAP1L4P1 ( Supplementary Fig. 1 ). The second hit was with rs4845320 ( P =1.98 × 10 −10 ; odds ratio=4.25), which lies in an LD block of 150 kb at 1q21.3 ( Fig. 1c ) that contains a cluster of genes encoding late cornified envelope (LCE) proteins [10] . The third significantly associated SNP, rs3127214 ( P =1.84 × 10 −8 ; odds ratio=2.96), is located at the 5′ end of TAGAP ( Fig. 1d ), encoding T-cell activation RhoGTPase-activating protein [11] , in an LD block of 120 kb at 6q25.3. Figure 1: Genetic association with candidaemia. ( a ) Manhattan plot showing the genome-wide P values of association with candidaemia. The y axis represents the −log 10 P values of 118,989 SNPs and their chromosomal positions are shown on the x axis. The horizontal red line shows the genome-wide significant threshold of P <5 × 10 −8 . The P -values were obtained by logistic regression test after adjusting for the first four components from the multidimensional scaling analysis. Regional association plots at ( b ) 1p13.1, ( c ) 1q21.3 and ( d ) 6q25.3. The P values of genotyped SNPs are plotted as –log 10 values against their physical chromosomal positions (hg19). Estimated recombination rates from the 1000 Genomes European population show the local LD structure. Inset, the colours of the SNPs indicate LD with the top-associated SNPs according to a scale from r 2 =0 to r 2 =1 based on pairwise r 2 values from the 1000 Genomes European population. Lower panel, gene annotations from the University of California Santa Cruz genome browser (hg19). Full size image Table 1 Significantly associated loci with candidaemia that were validated using disease-matched controls. 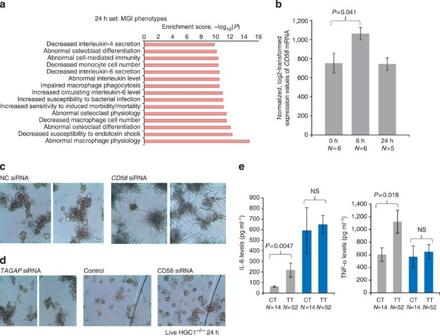Figure 2: Functional validation of CD58 in antifungal host denfense. (a) Common phenotype enrichment in the mouse using the Mouse Genome Informatics (MGI) phenotype data of the 93 genes differentially expressed at 24 h between control andCD58siRNA cells. (b)CD58gene expression levels in wild-type macrophages at 0, 6 and 24 h uponCandidainfection were extracted from the microarray experiment. (c) Human monocyte-derived macrophages were transfected with control and CD58 siRNA, respectively, for 48 h. Macrophages were co-incubated with liveC. albicansfor an additional 24 h. Representative microscopic photos of theCandidaoutgrowth through the macrophage are shown. The magnification is × 40. (d) First panel: macrophages were transfected with control and TAGAP siRNA, respectively, for 48 h. Macrophages were co-incubated with liveC. albicansfor an additional 24 h. Second panel: control and CD58 siRNA-transfected macrophages were co-incubated with liveC. albicans Δhgc1strain for an additional 24 h. Representative microscopic photos of theCandidaoutgrowth through the macrophage are shown. (e) Human monocyte-derived macrophages from 66 healthy volunteers with differentCD58SNP rs12025416 genotypes were stimulated withCandidafor 24 h (grey bars) or with LPS for 24 h (blue bars), and the supernatant was collected for IL-6 and TNF-α measurements. Average values ofCandida-induced IL-6 levels among CT individuals is 62.68 and among TT is 218.19; whereas for LPS it is 592.71 in CT group and 650.26 in TT group. Average values ofCandida-induced TNF-α levels among CT individuals is 603.57 and among TT is 1,122.88; whereas for LPS it is 570.02 in CT group and 648.36 in TT group. The error bars indicate s.e.m.. The correlation between cytokine production and genotypes was tested by the Wilcoxon rank sum test. NS; not significant. Full size table Validation and replication of three associated SNPs Since we used a large population-based control cohort for discovering candidaemia susceptibility loci, we tested whether these associations could be confirmed using 146 disease-matched controls ( Table 2 ). We observed a significant difference between cases and controls at two loci ( LCE4A-C1orf68 and TAGAP ), whereas at the CD58 locus we observed a trend of association ( Table 1 ). This latter effect could be explained by the small number of controls and/or low frequency of the risk allele at rs17035850 ( Table 1 ). The top CD58 SNP (rs17035850) is a rare variant with a minor allele frequency (MAF) of 0.012, and the second CD58 SNP (rs12025416) is a frequent one with MAF of 0.13. We assessed the pairwise LD between these two CD58 SNPs in our population-based controls. We observed both a low correlation ( r 2 =0.09) and a high D′ (D′>0.96) between these two SNPs, indicating the existence of rare risk haplotype that carry the risk alleles of these two SNPs. Therefore, we also tested for association at the second CD58 top SNP, rs12025416, which is more frequent, and we observed a significant association with susceptibility to candidaemia ( P =0.022). Therefore, these results suggest that the observed associations are true genetic associations. Table 2 Clinical characteristics of the candidaemia cohort. Full size table To further evaluate these associations genetically, we carried out replication analysis by genotyping the four SNPs in two independent candidaemia cohorts (one of 75 African-American patients and one of 27 European patients from Switzerland). Because of the small size of these additional cohorts, we found no successful replication in two independent cohorts, although we observed only a trend of association for rs4845320 SNP in the TAGAP locus in the African-American cohort ( Supplementary Table 1 ). Since the Swiss candidaemia replication cohort included matched controls, we performed a joint analysis of the discovery cohort with the matched controls and the Swiss candidaemia replication cohort. This analysis revealed an improved association for two loci: rs12025416 in the CD58 locus ( P =0.015) and rs4845320 in the LCE4A - C1orf68 locus ( P =0.0036), with the same allelic direction and without any evidence for heterogeneity between the two cohorts ( Supplementary Table 2 ). Functional annotation of candidaemia-associated SNPs To understand how the candidaemia-associated SNPs from these three loci affect disease, we intersected the three top SNPs as well as their proxies ( r 2 ≥0.8 and D′=1) with functional information from ENCODE using HaploReg [12] . 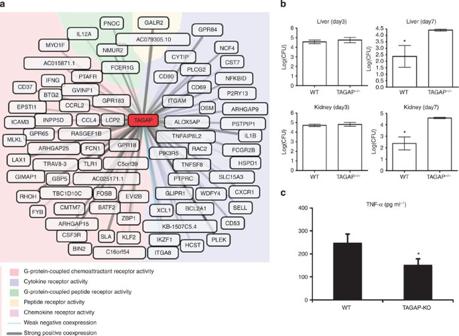Figure 3: Functional validation of TAGAP in antifungal host denfense. (a) The co-expression analysis (GeneNetwork) to predict the potential role of TAGAP. Coexpressed genes are coloured based on their gene ontology molecular function. (b) Wild-type and Tagap−/−mice were infected intravenously withC. albicansblastoconidia (5 × 105CFU per mouse). Subgroups of animals were killed on days 3 and 7 of infection, and fungal outgrowth was assessed in both liver (upper panel) and kidneys (lower panel). The results are pooled data from at least five mice per group (mean±s.e.m.). (c) Splenocytes isolated from wild-type and Tagap−/−mice were stimulated withC. albicansfor 24 h, after which TNF-α was measured by enzyme-linked immunosorbent assay in the supernatant (mean±s.e.m.). We found 7, 19 and 5 SNPs to be in high LD with rs17035850, rs4845320 and rs3127214 SNPs, respectively ( Supplementary Table 3 ). All SNPs that were in LD with the three candidaemia top SNPs were located in non-coding regions and not within exons of protein-coding genes. Some of these SNPs were overlapping with ENCODE-characterized regulatory regions, such as enhancers and/or DNase hypersensitive sites, suggesting that these SNPs may regulate gene expression. Next, we tested whether these SNPs affect expression of nearby genes using publicly available blood expression quantitative trait locus data from 5,000 samples [13] . However, we found no significant expression quantitative trait loci for these SNPs. Thus, it could be that the identified SNPs are likely in LD with regulatory variants, but these may only be functional in cell types such as macrophages and under stimulatory conditions with Candida infection. This will be important to test in the future studies. Interestingly, the LD block around the top-associated SNP, rs17035850, contains not only the CD58 protein-coding gene, but also non-coding genes, namely RP5-1086K13.1 , RP4-655J12.4 and the pseudogene NAP1L4P1 ( Supplementary Fig. 1 ). Since many lncRNAs are co-regulated with their protein-coding gene in cis , there is a possibility that RP5-1086K13.1 lncRNA is co-regulating CD58 . To test this possibility, we extracted all co-regulated genes with RP5-1086K13.1 using the GeneNetwork database [14] . We found that RP5-1086K13.1 is significantly co-regulated with CD58 compared with all other genes in the human genome ( Supplementary Table 4 ). This observation suggests the possibility that even if the SNP affects the expression of RP5-1086K13.1, that may in turn affect CD58 expression levels. Association of CD58 and TAGAP SNPs with severity of disease In addition to increasing susceptibility to candidaemia, the polymorphisms identified above may also influence the severity of the disease. Indeed, assessment of the effect of these SNPs revealed that CD58 SNP rs17035850 associated with persistent fungemia, defined as positive blood cultures for >5 days despite adequate therapy ( P =0.005), while TAGAP SNP rs3127214 associated with disseminated disease in the organs (P =0.017) (see also Supplementary Table 5 ). The transcriptomes of CD58- and TAGAP-deficient macrophages Practically nothing is known regarding the roles of CD58 and TAGAP in antifungal host defence. To identify the antifungal host defence mechanisms influenced by these two genes, we assessed genome-wide transcriptional changes in wild-type macrophages, as well as macrophages in which the expression of CD58 and TAGAP was strongly reduced by small interfering RNA (siRNA) transfection at 6 and 24 h upon Candida infection. Efficient downregulation of CD58 messenger RNA (mRNA) was obtained by siRNA transfection, whereas only a mild effect was seen on TAGAP mRNA levels ( Supplementary Fig. 2 ). Genome-wide transcriptional changes in wild-type and CD58-deficient macrophages showed a total of 169 (at 6 h) and 93 (at 24 h) transcripts with at least a 1.25-fold differential expression ( Supplementary Fig. 3 ). Enrichment analysis showed that the differentially expressed genes are enriched for innate immune function, regulation of cytokine production and general cellular responses to bacterial infections ( Supplementary Fig. 4 ). Furthermore, we investigated whether mutations in these differentially expressed genes show any common phenotypes in the mouse using the Mouse Genome Informatics phenotype data integrated in the GeneNetwork database. Indeed, we observed a significant enrichment for genes in which mutations may cause altered levels of IL-6 and tumor necrosis factor (TNF)-α secretion, and impaired macrophage phagocytosis ( Fig. 2a ). These data suggest that altered expression levels of CD58 may regulate Candida phagocytosis on one hand, and indirectly regulate IL-6 and TNF-α secretion on the other hand. Figure 2: Functional validation of CD58 in antifungal host denfense. ( a ) Common phenotype enrichment in the mouse using the Mouse Genome Informatics (MGI) phenotype data of the 93 genes differentially expressed at 24 h between control and CD58 siRNA cells. ( b ) CD58 gene expression levels in wild-type macrophages at 0, 6 and 24 h upon Candida infection were extracted from the microarray experiment. ( c ) Human monocyte-derived macrophages were transfected with control and CD58 siRNA, respectively, for 48 h. Macrophages were co-incubated with live C. albicans for an additional 24 h. Representative microscopic photos of the Candida outgrowth through the macrophage are shown. The magnification is × 40. ( d ) First panel: macrophages were transfected with control and TAGAP siRNA, respectively, for 48 h. Macrophages were co-incubated with live C. albicans for an additional 24 h. Second panel: control and CD58 siRNA-transfected macrophages were co-incubated with live C. albicans Δhgc1 strain for an additional 24 h. Representative microscopic photos of the Candida outgrowth through the macrophage are shown. ( e ) Human monocyte-derived macrophages from 66 healthy volunteers with different CD58 SNP rs12025416 genotypes were stimulated with Candida for 24 h (grey bars) or with LPS for 24 h (blue bars), and the supernatant was collected for IL-6 and TNF-α measurements. Average values of Candida -induced IL-6 levels among CT individuals is 62.68 and among TT is 218.19; whereas for LPS it is 592.71 in CT group and 650.26 in TT group. Average values of Candida -induced TNF-α levels among CT individuals is 603.57 and among TT is 1,122.88; whereas for LPS it is 570.02 in CT group and 648.36 in TT group. The error bars indicate s.e.m.. The correlation between cytokine production and genotypes was tested by the Wilcoxon rank sum test. NS; not significant. Full size image Functional validation of CD58 for anti-Candida host defence We next tested the CD58 mRNA levels in macrophages at 6 and 24 h upon Candida infection using microarray data. We observed a significant upregulation of CD58 in response to Candida infection at 6 h ( Fig. 2b ; P =0.04), whereas no difference was seen at 24 h, suggesting CD58 as an early-response gene in host defence against Candida . To validate the functional role of CD58 in anti- Candida response further, we investigated the phenotypes of macrophages with silenced CD58. It has been demonstrated that yeast-to-hyphae transition is one of the virulence factors for Candida to escape macrophage phagocytosis [15] . As expected, live Candida through germ-tube formation could escape macrophage phagocytosis in the control siRNA-transfected group, as well as in the TAGAP siRNA group. Strikingly, a massive fungal outgrowth with extensive fungal hyphae formation was observed in the CD58 siRNA-transfected group ( Fig. 2c ), showing that CD58 is important for Candida phagocytosis and inhibition of germination. To validate this possibility further, the co-localization of CD58 and Candida in the phagosome was examined by fluorescence microscopy. Upon Candida phagocytosis, a clear recruitment of CD58 (green) around the calcofluor white-labeled Candida (blue) was observed, indicating co-localization of CD58 and Candida during phagocytosis ( Supplementary Fig. 5 ). When a yeast-locked Δ hgc 1 C. albicans strain was used, there was no defect in the control of fungal growth in cells transfected with CD58 siRNA ( Fig. 2d ). As the transcriptome and pathway analyses in CD58-deficient macrophages implicated altered levels of IL-6 and TNF-α secretion, we tested the role of CD58 SNPs with these cytokine levels. The cytokines IL-6 and TNF-α were quantified from macrophages stimulated with either lipopolysaccharide (LPS) or Candida . The top CD58 SNP, rs17035850, is a rare SNP with very low risk allele frequency. Therefore, we tested the second CD58 top SNP, rs12025416, which occurs more frequently, for association with cytokine levels. Functional genetic validation showed that CD58 SNP rs12025416 genotypes modulated cytokine production, where the risk allele C was associated with lower levels of Candida -stimulated IL-6 and TNF-α ( Fig. 2e , P =0.0047 and P =0.018, respectively). In contrast, we found no association with LPS-stimulated IL-6 and TNF-α levels ( Fig. 2e ), confirming the specific role of CD58 polymorphisms in response to Candida infection. Functional validation of TAGAP for anti-Candida host defence Because TAGAP siRNA inhibition in primary macrophages was not efficient, we interrogated the GeneNetwork database to predict TAGAP function based on co-expression data extracted from ~80,000 Affymetrix microarray experiments (see www.genenetwork.nl/genenetwork ). Several gene ontology molecular functions, such as chemoattractant receptor activity and cytokine production, were strongly influenced by TAGAP ( Fig. 3a ). To validate these pathways, the role of TAGAP was tested in an in vivo disseminated candidiasis model in Tagap- deficient mice. While the fungal loads did not differ between control and knockout mice early during infection, the Tagap −/− mice were incapable of clearing the fungus from organs at the later stages of infection ( Fig. 3b ). In addition, splenocytes isolated from Tagap −/− mice produced significantly less TNF-α compared with control animals ( Fig. 3c ). Figure 3: Functional validation of TAGAP in antifungal host denfense. ( a ) The co-expression analysis (GeneNetwork) to predict the potential role of TAGAP. Coexpressed genes are coloured based on their gene ontology molecular function. ( b ) Wild-type and Tagap −/− mice were infected intravenously with C. albicans blastoconidia (5 × 10 5 CFU per mouse). Subgroups of animals were killed on days 3 and 7 of infection, and fungal outgrowth was assessed in both liver (upper panel) and kidneys (lower panel). The results are pooled data from at least five mice per group (mean±s.e.m.). ( c ) Splenocytes isolated from wild-type and Tagap −/− mice were stimulated with C. albicans for 24 h, after which TNF-α was measured by enzyme-linked immunosorbent assay in the supernatant (mean±s.e.m.). Full size image This first genome-wide association study assessing genetic susceptibility to a fungal infection identified three novel risk factors for susceptibility to candidaemia, namely CD58 , the LCE4A-C1orf68 locus and TAGAP . Carrying two or more risk alleles from these loci increases the risk for candidaemia by >19-fold ( Supplementary Fig. 6 ). Using transcriptomic analysis and immunological validation, we identified unknown roles of CD58 and TAGAP in host defence against Candida species. Genetic association studies are extremely challenging in systemic fungal infections owing to the inherent difficulty of the relatively low number of patients available. The difficulty of enrolling a large number of candidaemia patients is exemplified by the fact that earlier cohorts had no more than 60 patients [16] , [17] . To surpass these difficulties, we took several steps. First, we increased the number of patients by combining patients of European descent from Duke University and Radboud University Nijmegen Medical Center. Second, for the discovery analysis we used a large cohort of 11,920 population-based controls. Analysing a large number of population-based controls against a small number of cases could potentially yield spurious associations owing to population substructure. Therefore, we strictly relied on confirming the significant findings by comparing the patients with the underlying disease-matched control cohort. Additional validation studies were performed in independent cohorts. Third, we focused on genes and gene regions known to be involved in immune-mediated diseases by using the Immunochip array. Finally, we confirmed the biological significance of our findings by immunological and functional genomics experiments. Our findings have important implications. On one hand, the 19-fold increased risk of developing candidaemia in individuals carrying two or more risk alleles opens the possibility of using these SNPs to classify at-risk patients, and identify individuals who could benefit from prophylactic antifungal treatment. On the other hand, we have identified novel pathways of host defence mechanisms against fungi that contribute to a better understanding of host defence, and which may also be used for designing future immunotherapeutic strategies. In this respect, the unexpected identification of CD58 as an important factor mediating Candida phagocytosis and the inhibition of germination on one hand, and modulation of Candida- specific cytokine production on the other hand, is an important step towards understanding the pathogenesis of the infection. CD58 is known as a member of the immunoglobulin superfamily [18] and mediates adhesion and activation of T lymphocytes [19] . It has been shown to be involved in the host defence against viral infections, such as hepatitis B [20] . The role identified here in inhibiting fungal germination at the level of the phagosome is unexpected and sheds light on a novel function of this molecule. The role of the LCE4A-C1orf68 locus for anti- Candida host defence could have been anticipated from its involvement in the barrier function of the epithelium, as Candida colonization of the mucosae is one of the main risk factors for candidaemia in at-risk patients [21] . In contrast, nothing was known regarding a potential role for TAGAP in antifungal host defence. Using a GeneNetwork microarray database and co-expression analysis, and immunological validation in mice with a genetic defect in Tagap , we demonstrate its role in Candida -induced inflammation and antifungal host defence. Interestingly, the genes we have identified as being involved in the susceptibility to candidaemia are also involved in the genetic susceptibility to immune-mediated diseases. Polymorphisms in CD58 have been reported to increase susceptibility to multiple sclerosis [22] and rheumatoid arthritis [23] , LCE4A-C1orf68 locus variants are associated with rheumatoid arthritis [24] and psoriasis [25] and TAGAP polymorphisms influence several autoinflammatory diseases [23] , [26] , [27] , [28] , [29] . These data point to strong similarities between the immune-mediated mechanisms involved in the host defence against fungal pathogens and those for immune-mediated pathology. This hypothesis is strengthened by the associations described between anti- Candida -specific antibodies and Crohn’s disease [30] . Similar shared relationships have been proposed for other pathologies such as leprosy and Crohn’s disease [28] , and it has even been hypothesized that the genetic susceptibility to autoimmune diseases in modern human populations was shaped by evolutionary pressure exerted by infections [31] , [32] . In conclusion, this first, unbiased, genetic association study in a fungal infection demonstrates the potential of functional genomics approaches to identify novel risk factors in infections even in clinical conditions, in which a limited number of patients are available. Our study highlights genetic variants in three novel antifungal host defence mechanisms that increase susceptibility to candidaemia. Discovery cohort Adult candidaemia patients were enrolled after informed consent at the Duke University Hospital (DUMC, Durham, North Carolina, USA) and Radboud University Nijmegen Medical Centre (Nijmegen, The Netherlands). Disease-matched controls were enrolled after informed consent at the Duke University Hospital (DUMC). The study was approved by the institutional review boards ( Supplementary Table 6 ) at each study centre, and enrollment occurred between January 2003 and January 2009 (refs 33 , 34 ). Patients must have had at least one positive blood culture for a Candida species. A total of 217 patients of European ancestry (36 of the Netherlands origin and 181 of USA origin) were included in the study (for clinical characteristics, see Table 2 ). Two different control groups were employed. One, consisting of 11,920 population-based individuals of European ancestry [26] , [35] , was used for the discovery phase of the study. The second control group consisted of 146 candidiasis-free but otherwise matched patients. Non-infected patients were recruited from the same hospital wards as infected patients so that co-morbidities and clinical risk factors for infection were similar. This second control group was used to confirm the candidate SNPs identified in the discovery phase. The infected subjects at DUMC were followed prospectively for up to 12 weeks following diagnosis of candidaemia to determine their clinical outcome. Disseminated infection was defined as the presence of Candida species at normally sterile body sites other than the bloodstream or urine. Persistent fungemia was defined as ≥5 days of persistently positive blood cultures. Validation cohorts Two independent cohorts of patients with candidaemia were used for validation studies. First, a cohort of 75 patients of African-American descent with candidaemia was recruited at DUMC, and 54 patients of African-American descent without candidaemia from the same wards served as a disease-matched control group. Second, a cohort of 69 European surgical intensive care unit patients, including 29 cases of invasive candidiasis (without candidaemia) and 40 non-infected controls, were recruited for the Funginos study, as described elsewhere [36] . Genotyping and quality control The case and the control samples of the discovery cohort were genotyped using the Immunochip according to Illumina’s protocols [26] . We applied SNP quality-control filters to exclude SNPs with (a) a low call rate (<99%), (b) a Hardy–Weinberg equilibrium of P <0.01 in control samples only and (c) a MAF of <0.01. In the end, 118,989 SNPs were used for case-control analysis. We also excluded 54 samples with a low genotyping rate (<98%) and 40 ethnic outlier samples based on multidimensional scaling analysis ( Supplementary Fig. 7 ) [35] . We included 217 candidaemia cases and 11,920 controls of Caucasian descent in the discovery phase of the case-control association analysis. The replication cohorts were genotyped at four SNPs using the Competitive Allele-Specific PCR (KASP) system according to the manufacturer’s protocol (LGC Genomics; http://www.lgcgenomics.com , formerly KBioscience). The KASP allele-specific forward primers and common reverse primer were designed by Kraken assay design and workflow management software (LGC Genomics, formerly KBioscience). Results were analysed on KlusterKaller software (LGC Genomics, formerly KBioscience) according to standard protocols and quality controls. Statistical analysis In the discovery phase, the associations between Immunochip SNPs and candidaemia susceptibility were tested by logistic regression after adjusting for the first four components from the multidimensional scaling analysis using PLINKv1.07 (ref. 37) [37] . A strong inflation in Immunochip studies has been observed, as the selection of SNPs is biased towards only loci associated with immune-mediated traits [26] . Therefore, we considered SNPs that map to non-immune regions but are present on the Immunochip to calculate the inflation factor. Comparison of the genetic inflation factor of all SNPs ( λ =1.22) with the genetic inflation factor of non-immune SNPs ( λ =1.102) indicated that there was little population stratification effect ( Supplementary Fig. 8 ). We considered P <5 × 10 −8 as the threshold for significant association. The association to the top-associated SNPs within the validation and replication cohorts was tested using the Cochran–Armitage trend test, and meta-analysis was conducted using the Mantel–Haenszel method. Heterogeneity across the two cohorts was examined using the Breslow–Day test. We tested the cumulative effects of three risk SNPs on candidaemia risk among individuals carrying either 1 or 2 and more risk alleles. The odds ratios were calculated relative to the individuals with no risk alleles for the three SNPs. CD58/TAGAP knockdown and phagocytosis experiments Human monocyte-derived macrophages were obtained by first allowing peripheral blood mononuclear cells to adhere to the plate for 90 min and the non-adherent cells were washed away by phosphate-buffered saline. The remaining adherent monocytes were differentiated into macrophages by incubating with RPMI containing M-CSF (50 ng ml −1 ) and 10% human pooled serum for 6 days [38] . Macrophages from five different volunteers were transfected with CD58 siRNA (L-004538-00-0005), TAGAP siRNA (L-008711-01-0005) or control siRNA (D-001810-10-20) by Dharmafect 4 for 2 days (Thermo Scientific). Total RNA was isolated at 6 and 24 h, and global gene expression was profiled using an Illumina Human HT-12 Expression BeadChip [39] . Differentially expressed genes by at least 1.25-fold between control and CD58 siRNA cells were subjected to pathway enrichment analysis using GeneNetwork analysis [14] . After siRNA transfection, macrophages were exposed to live C. albicans at multiplicity of infection of 1 for 24 h, after which the phagocytosis and fungal outgrowth was determined by microscopy. The role of fungal germination was assessed using the yeast-locked Hgc1 -deficient C. albicans strain (provided by Dr Bernhard Hube, Jena University). Cytokine concentrations were determined by enzyme-linked immunosorbent assay. In vitro macrophage stimulation assays The effect of SNPs in CD58 on cytokine production was studied in monocyte-derived macrophages isolated from a cohort of 66 healthy Europeans. Macrophages were incubated at 37 °C for 24 h with RPMI culture medium, LPS (10 ng ml −1 , Sigma-Aldrich, MO, USA), or heat-killed C. albicans yeasts or hyphae (1 × 10 6 microorganisms per ml). Cytokines were measured using an enzyme-linked immunosorbent assay (R&D Systems, MN, USA), and the correlation between cytokine production and genotypes was tested by the Wilcoxon rank sum test. Systemic C. albicans infection in TAGAP-deficient mice C57BL/6J and Tagap loss-of-function female mice [40] , [41] (8–12 weeks) were used for assessing their susceptibility to C. albicans. The Tagap −/− mouse was reported in the original publication by Bauer et al. [40] , the accession number for the gene targeted in this knockout model is NM_145968, which corresponds to the Tagap gene. However, Bauer et al. [40] refer to this gene as Tagap1 . To clarify the gene targeted in these mice, we developed a quantitative reverse transcriptase-PCR method and showed that the targeted mice lacked Tagap mRNA, consistent with the accession number referenced in the original publication. See also MGI ID 3615484 for gene information and MGI ID 3603008 for mouse strain information. The experiments were approved by the Ethics Committee on Animal Experiments of the University of Athens. Mice were injected with live C. albicans blastoconidia 5 × 10 7 CFU per mouse. The fungal loads in the liver and kidneys were assessed by microbiological dilution plating on days 3 and 7 after infection. Cytokine production capacity was assessed after stimulation of splenocytes (1 × 10 5 per well) with C. albicans (1 × 10 6 microorganisms per well). How to cite this article: Kumar, V. et al. Immunochip SNP array identifies novel genetic variants conferring susceptibility to candidaemia. Nat. Commun. 5:4675 doi: 10.1038/ncomms5675 (2014).